Prompt meningeal reconstruction mediated by oxygen-sensitive AKAP12 scaffolding protein after central nervous system injury The meninges forms a critical epithelial barrier, which protects the central nervous system (CNS), and therefore its prompt reconstruction after CNS injury is essential for reducing neuronal damage. Meningeal cells migrate into the lesion site after undergoing an epithelial–mesenchymal transition (EMT) and repair the impaired meninges. However, the molecular mechanisms of meningeal EMT remain largely undefined. Here we show that TGF-β1 and retinoic acid (RA) released from the meninges, together with oxygen tension, could constitute the mechanism for rapid meningeal reconstruction. AKAP12 is an effector of this mechanism, and its expression in meningeal cells is regulated by integrated upstream signals composed of TGF-β1, RA and oxygen tension. Functionally, AKAP12 modulates meningeal EMT by regulating the TGF-β1-non-Smad-SNAI1 signalling pathway. Collectively, TGF-β1, RA and oxygen tension can modulate the dynamic change in AKAP12 expression, causing prompt meningeal reconstruction after CNS injury by regulating the transition between the epithelial and mesenchymal states of meningeal cells. The meninges is a membrane that covers central nervous system (CNS) tissue and is a complex structure composed of three distinct layers: the dura mater, the arachnoid membrane and the pia mater [1] . Functionally, the meninges are essential for CNS protection. In particular, cerebrospinal fluid (CSF), which fills the subarachnoid space, acts as a cushion preserving the CNS against mechanical impact and providing immunological defence [2] . Furthermore, arachnoid cells, present in the arachnoid membrane, exhibit epithelial cell properties and express high levels of tight junction proteins, which provide strong cell–cell adhesion to block the flow of materials [1] , [3] . Therefore, the arachnoid membrane functions as a meningeal barrier maintaining CNS homeostasis by selectively controlling the inflow of substances and immune cells from the external environment [4] . Meningeal barrier damage is commonly observed in various types of CNS injuries, such as brain trauma and spinal cord injury. Some accident patients can exhibit insufficient meningeal recovery after medical treatments, which can lead to CSF leakage, intracerebral aerocele, meningitis and extended secondary damage, thus resulting in an increased risk of death and permanent disability [5] , [6] . Consequently, the prompt reconstruction of an impaired meningeal barrier is crucial for reducing any additional neuronal damage after CNS injury. Following injuries to various tissues, epithelial cells, activated by epithelial–mesenchymal transition (EMT), migrate to the site of the lesion during an early stage of repair. Migratory epithelial cells are stabilized by mesenchymal–epithelial transition (MET), hence reconstructing the epithelium at a later stage in repair [7] . Although regulation of the transition between epithelial and mesenchymal states is thought to be essential for restoration of the meninges as well [8] , the molecular mechanisms of meningeal repair remain largely undefined. The meninges maintain high levels of transforming growth factor-beta 1 (TGF-β1) under normal conditions in adults [9] , [10] . As TGF-β1 is a major EMT-inducing factor [11] , it seems paradoxical that TGF-β1 is highly expressed in the meninges that acquire epithelial cell properties for proper barrier function. Therefore, it is of interest how the normal meninges retain epithelial properties despite the presence of TGF-β1. In addition, the meninges strongly express retinaldehyde dehydrogenase 2 (RALDH2), which is responsible for retinoic acid (RA) synthesis [12] , [13] . RA is a small lipophilic molecule, which acts through nuclear RA receptors (RARs), and has various effects on development, physiology and disease [14] , [15] , [16] . Several previous studies suggest that crosstalk between TGF-β isoforms and retinoids can have synergistic or antagonistic effects on development, neoplasia and the immune system [16] , [17] . Although TGF-β1 and RA expression is spatially correlated in the meninges, suggestive of crosstalk, their function in meningeal homeostasis during adulthood is unclear. The CNS occupies ~2% of total body mass, consumes 20% of the body’s oxygen and is well vascularized [18] , suggesting that the CNS has a high oxygen demand for its function and homeostasis. Thus, CNS tissue immediately remodels new vessels near the lesions through angiogenesis to overcome hypoxic conditions induced by vessel damage; consequently, oxygen concentrations are dynamically modulated during the repair process. Such alterations in oxygen tension are expected to regulate the expression of key molecules involved in meningeal reconstruction. However, the target molecules and their regulatory mechanisms during meningeal restoration are unknown. Expression of AKAP12, known as SSeCKS in mice and gravin in humans, is independently regulated by three different promoters (α, β and γ). While the expression of AKAP12γ is restricted to the testis, AKAP12α/β are expressed in most tissues, and are thought to play a compensatory role [19] . AKAP12, a scaffolding protein, has multiple functions in various biological events. AKAP12 regulates the movement of paraxial mesodermal cells [20] , vessel integrity [21] and blood neural barrier differentiation [22] , [23] during development. As a tumour suppressor protein, suppression of AKAP12 induces prostatic hyperplasia in vivo [24] and increases cell invasiveness in vitro [25] . We recently reported that AKAP12-expressing cells form a physical barrier that surrounds lesions after CNS injury, and AKAP12 knockout (KO) mice exhibit barrier structure malfunctions and loss of tight junction complexes, resulting in extended inflammation and more severe tissue damage [26] . In the present study, following up on our previous work, we identified AKAP12 as an effector candidate that could potentially modulate meningeal reconstruction, the expression of which is regulated in the arachnoid cells by integrated upstream signals comprised of TGF-β1, RA and oxygen tension. AKAP12 can modulate the transition between the epithelial and mesenchymal states in arachnoid cells by regulating the TGF-β1-non-Smad-SNAI1 signalling pathway during meningeal reconstruction. Our findings provide further insights into the mechanisms of meningeal reconstruction to reduce additional neuronal damage after CNS injury. AKAP12 is expressed in arachnoid cells of the meninges To investigate AKAP12 expression in CNS tissue, a histological analysis was performed. We found that AKAP12 expression is remarkably high in the meninges relative to that of other brain regions ( Fig. 1a , left panel). The AKAP12 signal completely overlapped those of fibronectin [27] and ERTR7 (ref. 28) [28] , markers of meningeal cells ( Fig. 1a , right panel). 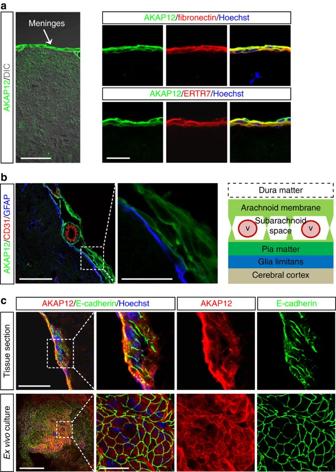Figure 1: AKAP12 is highly expressed in arachnoid cells that exhibit epithelial properties in the meninges. (a) AKAP12-positive cells are meningeal cells. Mouse brain sections were co-stained with antibodies against AKAP12 and meningeal cell markers (ERTR7 and fibronectin). Scale bar, 50 μm (left panel), 20 μm (right panels). (b) AKAP12-positive meningeal cells are meningeal arachnoid cells. Normal mouse brain sections were triple stained with antibodies against AKAP12, CD31 (a marker for endothelial cells) and GFAP (a marker for astrocytes). Scale bar, 50 μm (left panel), 20 μm (right panel). (c) AKAP12-positive meningeal cells highly express E-cadherin (a marker for arachnoid cells, a type of epithelial cell) in the normal meninges and inex vivo-cultured meningeal tissue. Scale bar, 50 μm (upper panel), 100 μm (lower panel), 20 μm (magnified panels). Each panel represents the results from independent experiments repeated at least five times using different animals or conditions. Figure 1: AKAP12 is highly expressed in arachnoid cells that exhibit epithelial properties in the meninges. ( a ) AKAP12-positive cells are meningeal cells. Mouse brain sections were co-stained with antibodies against AKAP12 and meningeal cell markers (ERTR7 and fibronectin). Scale bar, 50 μm (left panel), 20 μm (right panels). ( b ) AKAP12-positive meningeal cells are meningeal arachnoid cells. Normal mouse brain sections were triple stained with antibodies against AKAP12, CD31 (a marker for endothelial cells) and GFAP (a marker for astrocytes). Scale bar, 50 μm (left panel), 20 μm (right panel). ( c ) AKAP12-positive meningeal cells highly express E-cadherin (a marker for arachnoid cells, a type of epithelial cell) in the normal meninges and in ex vivo -cultured meningeal tissue. Scale bar, 50 μm (upper panel), 100 μm (lower panel), 20 μm (magnified panels). Each panel represents the results from independent experiments repeated at least five times using different animals or conditions. Full size image The arachnoid membrane is the middle layer of the meninges, between the dura and pia mater. The area between the arachnoid membrane and the pia mater is known as the subarachnoid space, a sponge-like structure containing vessel networks and trabeculae that extend from the arachnoid membrane [29] , [30] . As the connection between the dura mater and the arachnoid membrane is loose [31] , the dura mater is generally removed with skull when performing a brain extraction ( Fig. 1b , right graphics). The layer composed of AKAP12-positive cells in the meninges connected with the GFAP (glial fibrillary acidic protein)-positive glial limitans and formed a sheath around the meningeal vessels ( Fig. 1b ). Taken together with previous anatomical studies [30] , [32] , these data suggest that arachnoid cells, which form the arachnoid membrane and trabeculae, could be the main source of the AKAP12-positive cells. The pia mater is too thin to be easily distinguished from the trabeculae, which cover the pia mater; therefore, whether the pia mater expresses AKAP12 is unclear. Since arachnoid cells exhibit epithelial properties, including high expression of tight junction proteins [1] , [3] , we examined the expression of tight junction proteins in AKAP12-positive meningeal cells. As expected, immunohistochemical data showed that E-cadherin ( Fig. 1c , upper panel) and occludin ( Supplementary Fig. 1 , upper panel), epithelial cell markers, were highly expressed in AKAP12-positive meningeal cells. To observe AKAP12-positive cells in the meninges horizontally, we ex vivo cultured the meninges of postnatal day 3 mice. AKAP12-positive cells in the ex vivo -cultured meninges were densely packed with E-cadherin ( Fig. 1c , lower panel) and occludin ( Supplementary Fig. 1 , lower panel), similar to typical epithelial morphology. These results suggest that AKAP12 is highly expressed in arachnoid cells that have epithelial properties in the meninges. We attempted to use primary meningeal cells in a mechanistic study. However, commercial human primary meningeal cells did not exhibit epithelial properties ( Supplementary Fig. 2a,b ) and ex vivo -cultured mouse meningeal tissue lost most of its epithelial properties after 7 days of culture ( Supplementary Fig. 2c,d ). Since epithelial properties are necessary for mechanistic studies, we used ARPE-19 human retinal epithelial cells as a substitute experimental model. Since retinal tissue originates from the brain during development, and is part of the CNS, we thought that the properties of retinal epithelial cells would be more similar to those of the meninges rather than epithelial cells originating from other tissues. In addition, several key results obtained with ARPE-19 cells were confirmed with another cell line with epithelial properties, A549 cells ( Supplementary Fig. 3 ), implying that the mechanisms of AKAP12 are conserved in epithelial cells of various origins. TGF-β1 and RA induces high levels of AKAP12 expression Immunohistochemistry ( Fig. 2a ) showed that AKAP12, TGF-β1 and RALDH2 were strongly expressed in normal meninges. Because these parallel expression patterns could imply a correlation between TGF-β1 and RA and high levels of AKAP12, we examined whether TGF-β1 and RA regulate the expression of AKAP12 in vitro . Although RA increased AKAP12 messenger RNA expression in a dose-dependent manner, TGF-β1 had no effect on AKAP12 mRNA expression ( Fig. 2b,c ). Interestingly, TGF-β1 and RA co-treatment had a remarkable synergistic effect on the induction of AKAP12 compared with that of individual treatments ( Fig. 2b,c ). Co-treatment-induced AKAP12 expression occurred within 6 h and lasted for more than 48 h ( Fig. 2d ). These data explain how high levels of AKAP12 could be maintained in the meninges. 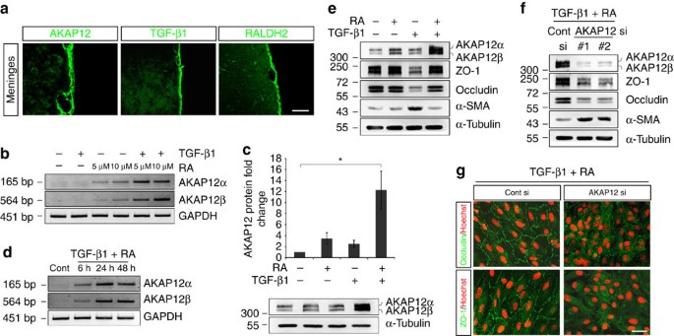Figure 2: A combination of TGF-β1 and RA induces high levels of AKAP12 expression, which maintains the epithelial properties of the meninges. (a) AKAP12 expression was co-localized with TGF-β1 and RALDH2 in the normal meningesin vivo. Scale bar, 40 μm (upper panels), 200 μm (lower panels). (b) ARPE-19 cells were serum starved for 24 h, and then treated with TGF-β1 (10 ng ml−1) and RA (5 and 10 μM) for 24 h. AKAP12 mRNA levels were markedly increased by co-treatment of these two factors compared with those of single treatments. (c) Co-treatment with TGF-β1 and RA synergistically increased AKAP12 protein levels. ARPE-19 cells were serum starved for 24 h, and then treated with TGF-β1 (10 ng ml−1) and RA (10 μM) for 24 h (mean±s.d.,n=4, analysis of variance followed by Tukey–Kramer test: *P=0.006). (d) Reverse transcription PCR was performed after treatment with TGF-β1 (10 ng ml−1) and RA (10 μM). AKAP12 mRNA levels were significantly increased after 6 h and were sustained up to 48 h. Glyceraldehyde-3-phosphate dehydrogenase was used as an internal control (Cont). (e) RA blocked TGF-β1-induced EMT. ARPE-19 cells were serum starved for 24 h, and then treated with TGF-β1 (10 ng ml−1) and RA (10 μM) for 48 h. (f) The inhibitory effect of RA on TGF-β1 was abolished in the absence of AKAP12. AKAP12 siRNA-transfected ARPE-19 cells were serum starved for 24 h and incubated in the presence of TGF-β1 (10 ng ml−1) and RA (10 μM) for 48 h. (g) Culture conditions were the same as inf. Cells on coverslips were fixed and immunostained with antibodies against occludin and ZO-1. Scale bar, 40 μm. Each panel represents the results from independent experiments repeated at least four times using different animals or conditions. Figure 2: A combination of TGF-β1 and RA induces high levels of AKAP12 expression, which maintains the epithelial properties of the meninges. ( a ) AKAP12 expression was co-localized with TGF-β1 and RALDH2 in the normal meninges in vivo . Scale bar, 40 μm (upper panels), 200 μm (lower panels). ( b ) ARPE-19 cells were serum starved for 24 h, and then treated with TGF-β1 (10 ng ml −1 ) and RA (5 and 10 μM) for 24 h. AKAP12 mRNA levels were markedly increased by co-treatment of these two factors compared with those of single treatments. ( c ) Co-treatment with TGF-β1 and RA synergistically increased AKAP12 protein levels. ARPE-19 cells were serum starved for 24 h, and then treated with TGF-β1 (10 ng ml −1 ) and RA (10 μM) for 24 h (mean±s.d., n =4, analysis of variance followed by Tukey–Kramer test: * P =0.006). ( d ) Reverse transcription PCR was performed after treatment with TGF-β1 (10 ng ml −1 ) and RA (10 μM). AKAP12 mRNA levels were significantly increased after 6 h and were sustained up to 48 h. Glyceraldehyde-3-phosphate dehydrogenase was used as an internal control (Cont). ( e ) RA blocked TGF-β1-induced EMT. ARPE-19 cells were serum starved for 24 h, and then treated with TGF-β1 (10 ng ml −1 ) and RA (10 μM) for 48 h. ( f ) The inhibitory effect of RA on TGF-β1 was abolished in the absence of AKAP12. AKAP12 siRNA-transfected ARPE-19 cells were serum starved for 24 h and incubated in the presence of TGF-β1 (10 ng ml −1 ) and RA (10 μM) for 48 h. ( g ) Culture conditions were the same as in f . Cells on coverslips were fixed and immunostained with antibodies against occludin and ZO-1. Scale bar, 40 μm. Each panel represents the results from independent experiments repeated at least four times using different animals or conditions. Full size image Because the meninges have strong epithelial properties required for separation of the CNS from the external environment, it is somewhat paradoxical that the meninges highly express TGF-β1, a major inducer of EMT. Similar to previous studies [11] , our in vitro data also showed that TGF-β1 induced typical EMT responses in two different epithelial cell lines, ARPE-19 ( Fig. 2e ) and A549 ( Supplementary Fig. 3a ). When the two cell lines were exposed to TGF-β1 for 48 h, levels of epithelial makers, including ZO-1 and occludin, were reduced, whereas α-SMA levels, a mesenchymal marker, were increased. Interestingly, we found that RA completely prevented the effects of TGF-β1, with highly increased levels of AKAP12 ( Fig. 2e ; Supplementary Fig. 3a ). To examine whether AKAP12 mediated the inhibition of TGF-β1 by RA, AKAP12-knockdown cells were co-treated with TGF-β1 and RA. Notably, the inhibitory effect of RA was abolished in the absence of AKAP12, and EMT occurred through TGF-β1 ( Fig. 2f,g ; Supplementary Fig. 3b,c ). These results suggest that the combination of TGF-β1 and RA induces high levels of AKAP12 expression, which maintains the epithelial properties of the meninges by inhibiting EMT despite the presence of TGF-β1. Oxygen modulates meningeal EMT/MET by regulating AKAP12 level To identify a correlation between AKAP12 expression and meningeal cell state during the reconstruction of the injured meninges, we examined serial expression of AKAP12 in meningeal cells after a focal brain injury induced by photothrombosis (PT). Under normal conditions, the meninges maintained high levels of AKAP12 expression ( Fig. 3a , left panels). On day 7 after injury, we observed that fibronectin (a marker for meningeal cells)-positive cells migrated from the meninges towards the lesion, implying that meningeal cells invaded the site of the lesion. AKAP12 levels were lower in migrating meningeal cells than in normal meninges ( Fig. 3a , middle panels). Interestingly, the proportion of AKAP12/fibronectin double-positive cells increased remarkably over time and most fibronectin-positive cells expressed high levels of AKAP12 on day 21 after injury ( Fig. 3a , right panels). In addition, α-SMA, a marker for motile cells that have mesenchymal properties, was not co-expressed with AKAP12 on day 7 after injury ( Fig. 3b ). Consistent with these data, when we analysed protein expression in lesional tissue by immunoblotting, AKAP12 had a similar expression pattern with that of the epithelial markers during the repair process; however, expression patterns of α-SMA were opposite to that of AKAP12 ( Fig. 3c ). These results show that AKAP12 expression was reduced in motile meningeal cells that had invaded into lesional tissue during the early stages of meningeal reconstruction and recovered as the cells became stationary during the later stages. 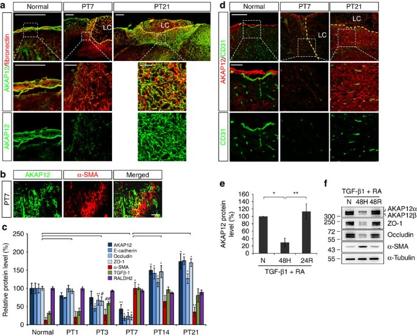Figure 3: Oxygen tension modulates the transition between epithelial and mesenchymal states during meningeal reconstruction by regulating AKAP12 expression. (a) AKAP12 levels were lower in meningeal cells invading into the lesional site than in the meninges. The number of AKAP12 and fibronectin double-positive cells increased over time. Scale bar, 200 μm (upper panels), 50 μm (magnified panels); LC, lesion core. (b) AKAP12 did not co-localize with α-SMA (a marker for motile mesenchymal cells). Scale bar, 40 μm. (c) AKAP12 expression was similar to that of epithelial markers in the repair process. Expression patterns of TGF-β1 and RA were not correlated with the dynamic changes in AKAP12 levels. Protein levels in lesional tissue extracts were determined by western blot analysis (mean±s.d.,n=3 mice per time point, analysis of variance (ANOVA) followed by Tukey–Kramer test: PT3_*P<0.0005, **P=0.039,#P=0.012,##P=0.047/PT7_*P<0.0005, **P=0.006/PT14_*P<0.0005/PT21_*P<0.0005, **P=0.001). (d) While intact vessels were well organized near the meninges under normal conditions, severe vessel damage was observed near the lesion on day 7 after injury. Neo-microvessels were generated in and near the scar tissue surrounding the lesion core on day 21 after injury. AKAP12 levels were dynamically regulated depending on the state of the vessels. Brain microvessels were stained with an antibody against CD31 (a marker for endothelial cells). Scale bar, 200 μm (upper panels), 50 μm (magnified panels); LC, lesion core. (e) AKAP12 expression was regulated by oxygen tension. After serum starvation for 24 h, ARPE-19 cells were exposed to hypoxic conditions for 48 h and then re-oxygenated for 24 h in the presence of RA (10 μM) and TGF-β1 (10 ng ml−1; mean±s.d.,n=4, ANOVA followed by Tukey–Kramer test: *P=0.002, **P=0.001). (f) Oxygen tension regulates AKAP12 and EMT marker expression in the presence of RA (10 μM) and TGF-β1 (10 ng ml−1). N, normoxia (21% oxygen); H, hypoxia (1% oxygen); R, reoxygenation (21% oxygen). Panelsa,b,d,frepresent the results from independent experiments repeated at least four times using different animals or conditions. Figure 3: Oxygen tension modulates the transition between epithelial and mesenchymal states during meningeal reconstruction by regulating AKAP12 expression. ( a ) AKAP12 levels were lower in meningeal cells invading into the lesional site than in the meninges. The number of AKAP12 and fibronectin double-positive cells increased over time. Scale bar, 200 μm (upper panels), 50 μm (magnified panels); LC, lesion core. ( b ) AKAP12 did not co-localize with α-SMA (a marker for motile mesenchymal cells). Scale bar, 40 μm. ( c ) AKAP12 expression was similar to that of epithelial markers in the repair process. Expression patterns of TGF-β1 and RA were not correlated with the dynamic changes in AKAP12 levels. Protein levels in lesional tissue extracts were determined by western blot analysis (mean±s.d., n =3 mice per time point, analysis of variance (ANOVA) followed by Tukey–Kramer test: PT3_* P <0.0005, ** P =0.039, # P =0.012, ## P =0.047/PT7_* P <0.0005, ** P =0.006/PT14_* P <0.0005/PT21_* P <0.0005, ** P =0.001). ( d ) While intact vessels were well organized near the meninges under normal conditions, severe vessel damage was observed near the lesion on day 7 after injury. Neo-microvessels were generated in and near the scar tissue surrounding the lesion core on day 21 after injury. AKAP12 levels were dynamically regulated depending on the state of the vessels. Brain microvessels were stained with an antibody against CD31 (a marker for endothelial cells). Scale bar, 200 μm (upper panels), 50 μm (magnified panels); LC, lesion core. ( e ) AKAP12 expression was regulated by oxygen tension. After serum starvation for 24 h, ARPE-19 cells were exposed to hypoxic conditions for 48 h and then re-oxygenated for 24 h in the presence of RA (10 μM) and TGF-β1 (10 ng ml −1 ; mean±s.d., n =4, ANOVA followed by Tukey–Kramer test: * P =0.002, ** P =0.001). ( f ) Oxygen tension regulates AKAP12 and EMT marker expression in the presence of RA (10 μM) and TGF-β1 (10 ng ml −1 ). N, normoxia (21% oxygen); H, hypoxia (1% oxygen); R, reoxygenation (21% oxygen). Panels a , b , d , f represent the results from independent experiments repeated at least four times using different animals or conditions. Full size image Since TGF-β1 and RA maintain high levels of AKAP12 in the normal meninges, we investigated whether dynamic changes in AKAP12 levels result from changes in TGF-β1 and RA expression during meningeal reconstruction. While AKAP12 had a biphasic pattern, gradually decreasing until day 7 after injury and then increasing from day 14, global levels of TGF-β1 were significantly increased from day 3 and were maintained until day 21. Global levels of RALDH2 remained constant during meningeal reconstruction ( Fig. 3c ). Likewise, expression patterns of TGF-β1 and RA did not correlate with the dynamic changes in AKAP12 levels, suggesting that a third factor regulates AKAP12 levels during meningeal reconstruction after CNS injury. During the early stage of most CNS injuries, hypoxic conditions accompany damaged microvessels near the lesion. This hypoxia induces angiogenesis and neo-microvessels resupply oxygen to the site of the lesion during later stages [33] , [34] . Furthermore, hypoxia is critical for induction of EMT, and affects various EMT factors through crosstalk [35] . Similar to other CNS injury models, our photothrombotic injury model also showed that brain microvessels were severely damaged after injury and new vessels formed near the lesional site during the later stages of repair. Under normal conditions, brain vessels were well organized near the meninges, which maintained high AKAP12 levels ( Fig. 3d , left panels), whereas vessels at the lesional site were severely damaged by day 7 after injury, and AKAP12 levels were significantly reduced in motile meningeal cells near the damaged vessels ( Fig. 3d , middle panels). On day 21 after injury, many newly formed vessels were apparent near the lesional site and AKAP12 levels were restored in the stationary meningeal cells, which formed the scar tissue surrounding the lesion ( Fig. 3d , right panels). Consistent with this data, global levels of AKAP12 in the lesional site were decreased on day 7 and highly increased on day 21 after injury in vivo ( Fig. 3c ). These data strongly suggest that oxygen tension is involved in the dynamic changes in AKAP12 expression, which depends on meningeal cell state during reconstruction. Therefore, we investigated the relationship between oxygen tension, AKAP12 levels and EMT in vitro . To imitate the high level of AKAP12 expression in the meninges, we performed in vitro assays in the presence of TGF-β1 and RA. When ARPE-19 cells were incubated under hypoxic conditions for 48 h in the presence of TGF-β1 and RA, AKAP12 expression was significantly reduced, but recovered following reoxygenation for 24 h ( Fig. 3e ). When we adjusted the expression of AKAP12 by changing oxygen concentrations, hypoxia induced EMT with decreased levels of AKAP12, while reoxygenation reversed this effect ( Fig. 3f ). These data suggest that oxygen concentrations can modulate the transition between epithelial and mesenchymal states by regulating AKAP12 levels in the presence of TGF-β1 and RA. Oxygen regulates the induction of AKAP12 by TGF-β1 and RA via RARβ Our results showed that TGF-β1, RA and oxygen tension comprise an integrated upstream signal that regulates the spatial and temporal response of AKAP12 during meningeal reconstruction after CNS injury ( Figs 2 and 3 ). Therefore, we investigated how oxygen tension regulates AKAP12 expression by intersecting with the TGF-β1 and RA pathways. Since induction of AKAP12 by TGF-β1 and RA was an immediate transcriptional response that occurred within several hours ( Fig. 2d ), we examined downstream transcription factors directly activated by TGF-β1 and RA. Although knockdown of Smad2 and RARα had no effect, Smad3 or/and RARβ knockdown specifically prevented TGF-β1- and RA-induced AKAP12 expression ( Fig. 4a ; Supplementary Fig. 4 ), suggesting that AKAP12 expression is directly regulated by the canonical pathways of TGF-β1 and RA [36] , [37] , and that activation of both Smad3 and RARβ is essential for maximal expression of AKAP12. However, the effect of Smad3 knockdown was less than that of RARβ, and there was no difference between RARβ single knockdown and Smad3/RARβ double knockdown ( P =1.000) ( Fig. 4a ; Supplementary Fig. 4 ). Therefore, the RA/RARβ pathway likely regulates AKAP12 induction, whereas the TGF-β1/Smad3 pathway is required for maximal expression of AKAP12. 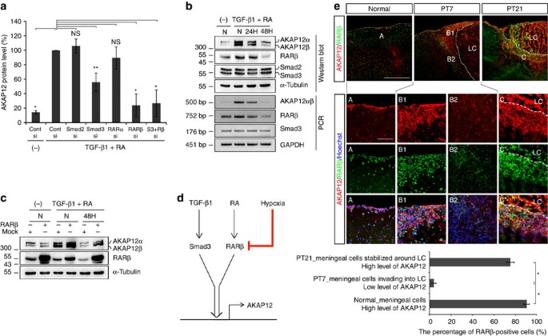Figure 4: Oxygen tension regulates induction of AKAP12 through TGF-β1 and RA at a transcriptional level via RARβ. (a) ARPE-19 cells were co-transfected with control (Cont), Smad2, Smad3, RARα and RARβ siRNA. Knockdown cells were treated with TGF-β1 (10 ng ml−1) and RA (10 μM) for 24 h after serum starvation for 24 h. Data are expressed relative to the control siRNA transfectant treated with TGF-β1 (10 ng ml−1) and RA (10 μM) for 24 h and are normalized to 100% (mean±s.d.,n=3, analysis of variance (ANOVA) followed by Tukey–Kramer test: *P<0.0005, **P=0.003; NS, not significant). (b) AKAP12 expression is reduced at a transcriptional level under hypoxia and correlates with RARβ expression. ARPE-19 cells were serum starved for 24 h and incubated under normoxia or hypoxia in the presence of TGF-β1 (10 ng ml−1) and RA (10 μM). (c) RARβ overexpression recovered the reduced level of AKAP12 under hypoxia. pCMV_flag human RARβ plasmid-transfected ARPE-19 cells were serum starved for 6 h and incubated under normoxia or hypoxia in the presence of TGF-β1 (10 ng ml−1) and RA (10 μM) for 48 h. (d) Diagram depicting the regulation of AKAP12 expression by hypoxia in the presence of TGF-β1 and RA. (e) Brain sections were co-stained with antibodies against AKAP12 and RARβ. AKAP12 expression has a similar pattern to that of RARβ during meningeal reconstruction. Scale bar, 500 μm (large panels), 100 μm (magnified panels). Three representative sections per mouse were analysed using Image J. Mean±s.d.,n=4 mice per time point, ANOVA followed by Tukey–Kramer test: *P<0.0005. N, normoxia (21% oxygen); H, hypoxia (1% oxygen); LC, lesion core. Panelsb,crepresent the results from independent experiments repeated at least four times. Figure 4: Oxygen tension regulates induction of AKAP12 through TGF-β1 and RA at a transcriptional level via RARβ. ( a ) ARPE-19 cells were co-transfected with control (Cont), Smad2, Smad3, RARα and RARβ siRNA. Knockdown cells were treated with TGF-β1 (10 ng ml −1 ) and RA (10 μM) for 24 h after serum starvation for 24 h. Data are expressed relative to the control siRNA transfectant treated with TGF-β1 (10 ng ml −1 ) and RA (10 μM) for 24 h and are normalized to 100% (mean±s.d., n =3, analysis of variance (ANOVA) followed by Tukey–Kramer test: * P <0.0005, ** P =0.003; NS, not significant). ( b ) AKAP12 expression is reduced at a transcriptional level under hypoxia and correlates with RARβ expression. ARPE-19 cells were serum starved for 24 h and incubated under normoxia or hypoxia in the presence of TGF-β1 (10 ng ml −1 ) and RA (10 μM). ( c ) RARβ overexpression recovered the reduced level of AKAP12 under hypoxia. pCMV_flag human RARβ plasmid-transfected ARPE-19 cells were serum starved for 6 h and incubated under normoxia or hypoxia in the presence of TGF-β1 (10 ng ml −1 ) and RA (10 μM) for 48 h. ( d ) Diagram depicting the regulation of AKAP12 expression by hypoxia in the presence of TGF-β1 and RA. ( e ) Brain sections were co-stained with antibodies against AKAP12 and RARβ. AKAP12 expression has a similar pattern to that of RARβ during meningeal reconstruction. Scale bar, 500 μm (large panels), 100 μm (magnified panels). Three representative sections per mouse were analysed using Image J. Mean±s.d., n =4 mice per time point, ANOVA followed by Tukey–Kramer test: * P <0.0005. N, normoxia (21% oxygen); H, hypoxia (1% oxygen); LC, lesion core. Panels b , c represent the results from independent experiments repeated at least four times. Full size image When ARPE-19 cells were exposed to hypoxic conditions after activation by co-treatment with TGF-β1 and RA, AKAP12 mRNA levels were decreased in a time-dependent manner, suggesting that oxygen tension regulates the expression of AKAP12 at a transcriptional level ( Fig. 4b ). As Smad3 and RARβ were associated with the induction of AKAP12 through TGF-β1 and RA, we investigated whether oxygen tension affects Smad3 and RARβ expression. While Smad3 expression was unchanged, oxygen concentrations regulated RARβ mRNA levels in a similar manner to those of AKAP12 ( Fig. 4b ). Furthermore, exogenously overexpressed RARβ recovered the reduction in AKAP12 induced by hypoxia ( Fig. 4c ), directly demonstrating that hypoxia blocks induction of AKAP12 through TGF-β1 and RA by reducing RARβ expression ( Fig. 4d ). Moreover, we examined the association between the expression of AKAP12 and that of RARβ after brain injury induced by photothrombosis. Under normal conditions, RARβ signals were strongly maintained in the nuclei of meningeal cells, which highly expressed AKAP12, and in neighbouring parenchymal cells near meninges ( Fig. 4e , panel A and graph), supporting previous reports that the meninges are the main source of RA [13] . On day 7 after injury, RARβ levels were significantly decreased in the invading meningeal cells in which AKAP12 levels were reduced ( Fig. 4e , panel B1,B2 and graph). As AKAP12 levels recovered by day 21, RARβ levels also increased ( Fig. 4e , panel C and graph). This in vivo data show that AKAP12 expression may be regulated according to the levels of RARβ, as shown in the in vitro data. Collectively, these results suggest that oxygen tension regulates AKAP12 induction through TGF-β1 and RA at a transcription level via RARβ. AKAP12 modulates EMT by regulating SNAI1 expression We explored the downstream mediators that enable AKAP12 to regulate the EMT response in our system. Since the effects of AKAP12 are not restricted to regulating specific proteins but also affect the general transition between epithelial and mesenchymal states, we focused on transcription factors that orchestrate EMT, such as SNAI1/2, Twist1/2 and ZEB1/2 (refs 38 , 39 ). When TGF-β1 signalling was blocked by RA, AKAP12 knockdown specifically upregulated SNAI1 expression ( Fig. 5a ; Supplementary Figs 3d and 5 ). Consistent with the AKAP12 suppression data in Fig. 2f,g , SNAI1 is a major TGF-β1-responsive transcriptional repressor that directly inhibits the transcription of E-cadherin and occludin [40] , [41] , and it also indirectly represses ZO-1 expression and upregulates α-SMA expression [42] , [43] . When RA blocked induction of SNAI1 through TGF-β1, AKAP12 expression patterns were opposite to those of SNAI1 ( Fig. 5b ). Furthermore, suppression of AKAP12 led to upregulation and nuclear translocation of SNAI1 when TGF-β1 was blocked by RA ( Fig. 5b,c ; Supplementary Fig. 3e ). Importantly, inhibition of SNAI1 completely blocked EMT induced by AKAP12 knockdown ( Fig. 5d ). Moreover, we examined the expression of endogenous SNAI1 at serial time points after brain injury induced by photothrombosis, and comparing this with that of normal brain. Immunostaining ( Fig. 5e ) showed that SNAI1 was not expressed in normal meningeal cells, which highly express AKAP12 ( Fig. 5e , panel A), and SNAI1 levels increased in invading meningeal cells in which AKAP12 levels were reduced on day 7 after injury ( Fig. 5e , panel B1,B2). On day 21, SNAI1 levels were reduced, concomitant with the recovery in AKAP12 ( Fig. 5e , panel C). Finally, we statistically confirmed that expression of SNAI1 was opposite to that of AKAP12 in vivo , similar to the in vitro data ( Fig. 5e , graph). These data suggest that AKAP12 modulates EMT by regulating the TGF-β1-SNAI1 signalling pathway. 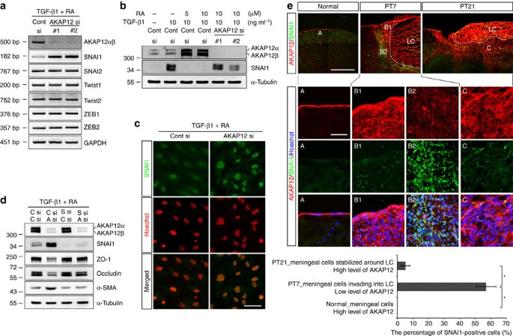Figure 5: AKAP12 modulates EMT by regulating SNAI1 expression. (a) AKAP12 knockdown specifically upregulated SNAI1 expression among all the EMT-inducing transcription factors analysed. ARPE-19 cells were transfected with two different siRNAs targeting AKAP12. Twenty-four hours after transfection, cells were serum starved for 6 h and then treated with TGF-β1 (10 ng ml−1) and RA (10 μM) for 24 h. (b) Expression of AKAP12 had the opposite pattern to that of SNAI1. Transfected ARPE-19 cells were serum starved for 24 h and then treated with TGF-β1 or/and RA for 24 h. (c) Suppression of AKAP12 led to nuclear translocation of SNAI1. Culture conditions were the same as inb(TGF-β1 (10 ng ml−1) and RA (10 μM)). Nuclei were stained with Hoechst 33342 (pseudocolored red). Scale bar, 20 μm. (d) Inhibition of SNAI1 completely blocked EMT induced by AKAP12 knockdown. Control (C), SNAI1 (S) and AKAP12 (A) siRNAs were co-transfected into ARPE-19 cells. Transfectants were serum starved for 24 h and incubated in the presence of TGF-β1 (10 ng ml−1) and RA (10 μM) for 48 h. (e) Brain sections were co-stained with antibodies against AKAP12 and SNAI1. Expression of AKAP12 had the opposite pattern to that of SNAI1 during meningeal reconstruction. Scale bar, 500 μm (large panels), 100 μm (magnified panels). Three representative sections per mouse were analysed using Image J. Mean±s.d.,n=4 mice per time point, analysis of variance followed by Tukey–Kramer test: *P<0.0005. LC, lesion core. Panelsa,b,c,drepresent the results from independent experiments repeated at least three times. Cont, control. Figure 5: AKAP12 modulates EMT by regulating SNAI1 expression. ( a ) AKAP12 knockdown specifically upregulated SNAI1 expression among all the EMT-inducing transcription factors analysed. ARPE-19 cells were transfected with two different siRNAs targeting AKAP12. Twenty-four hours after transfection, cells were serum starved for 6 h and then treated with TGF-β1 (10 ng ml −1 ) and RA (10 μM) for 24 h. ( b ) Expression of AKAP12 had the opposite pattern to that of SNAI1. Transfected ARPE-19 cells were serum starved for 24 h and then treated with TGF-β1 or/and RA for 24 h. ( c ) Suppression of AKAP12 led to nuclear translocation of SNAI1. Culture conditions were the same as in b (TGF-β1 (10 ng ml −1 ) and RA (10 μM)). Nuclei were stained with Hoechst 33342 (pseudocolored red). Scale bar, 20 μm. ( d ) Inhibition of SNAI1 completely blocked EMT induced by AKAP12 knockdown. Control (C), SNAI1 (S) and AKAP12 (A) siRNAs were co-transfected into ARPE-19 cells. Transfectants were serum starved for 24 h and incubated in the presence of TGF-β1 (10 ng ml −1 ) and RA (10 μM) for 48 h. ( e ) Brain sections were co-stained with antibodies against AKAP12 and SNAI1. Expression of AKAP12 had the opposite pattern to that of SNAI1 during meningeal reconstruction. Scale bar, 500 μm (large panels), 100 μm (magnified panels). Three representative sections per mouse were analysed using Image J. Mean±s.d., n =4 mice per time point, analysis of variance followed by Tukey–Kramer test: * P <0.0005. LC, lesion core. Panels a , b , c , d represent the results from independent experiments repeated at least three times. Cont, control. Full size image AKAP12 regulates SNAI1 via the non-Smad pathways of TGF-β1 To investigate how AKAP12 inhibits TGF-β1 signalling in the presence of RA, we identified the downstream pathways of TGF-β1 targeted by AKAP12. 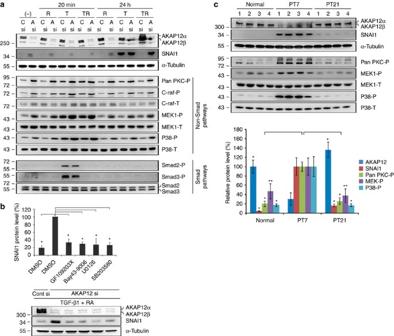Figure 6: AKAP12 regulates SNAI1 expression through the non-Smad pathways of TGF-β1. (a) AKAP12-knockdown cells were serum starved for 6 h and then treated with TGF-β1 (10 ng ml−1) and/or RA (10 μM) for 20 min and 24 h. Inhibition of AKAP12 activated the PKC/C-raf/MEK1 and p38 pathways among the examined non-Smad pathways of TGF-β1. Activation of these pathways was closely correlated with SNAI1 expression. This data represent the results from independent three experiments. R, RA; T, TGF-β1; TR, co-treatment of TGF-β1 and RA; C, Cont; A, AKAP12. (b) Specific inhibitors for PKC, C-raf, MEK1 and p38 blocked the upregulation of SNAI1 induced by AKAP12 knockdown. After serum starvation for 24 h, inhibitors were added to AKAP12-knockdown ARPE-19 cells treated with TGF-β1 (10 ng ml−1) and RA (10 μM) for 24 h (mean±s.d.,n=3, analysis of variance (ANOVA) followed by Tukey–Kramer test: *P<0.0005). GF 109203X (general PKC inhibitor): 5 μM, Bay 43-9006 (Raf-1 inhibitor): 1 μM, U0126 (MEK1 inhibitor): 10 μM, SB203580 (P38 inhibitor): 10 μM. (c) Lesional tissues from four mice per time point were collected and protein levels in the lesional tissue extracts were determined by western blot analysis. AKAP12 expression dynamically changed during the repair process. Phosphorylation of PKC, MEK1, p38 and SNAI1 expression had the opposite pattern to that of AKAP12 levels, similar to thein vitrodata. Bands were quantified with Image J. AKAP12, SNAI1 and pan-PKC-P densities were normalized to that of α-tubulin. The densities of MEK-P and p38-P were normalized to that of total MEK and total p38, respectively (mean±s.d.,n=4 mice per time point, ANOVA followed by Tukey–Kramer test: normal_*P<0.0005, **P=0.003/PT 21_*P<0.0005, **P=0.001). As shown in Figure 6a , both Smad and the non-Smad pathway were activated 20 min after single treatment with TGF-β1. Interestingly, Smad pathway activation by TGF-β1 was completely blocked by co-treatment with RA. However, activation of the protein kinase C (PKC)/C-raf/MEK1 and the p38 pathway by TGF-β1 was unaffected by RA. Furthermore, while Smad pathway activation by TGF-β1 was unchanged according to AKAP12 levels, AKAP12 inhibition activated the PKC/C-raf/MEK1 and p38 pathway following TGF-β1 treatment. Moreover, AKAP12 knockdown increased basal levels of SNAI1 and phosphorylation of PKC, C-raf, MEK and p38 even in the absence of TGF-β1. At 24 h after TGF-β1 and/or RA treatment, single treatment with TGF-β1 significantly increased SNAI1 levels, whereas single treatment with RA had no effect on SNAI1 expression. However, co-treatment with RA completely blocked SNAI1 induction by TGF-β1 (with high levels of AKAP12). Further, when induction of AKAP12 was blocked by short interfering RNA (siRNA), the inhibitory effect of RA on SNAI1 induction by TGF-β1 was neutralized, with concomitant phosphorylation of PKC, C-raf, MEK and p38. Finally, specific inhibitors for PKC, C-raf, MEK1 and p38 effectively blocked AKAP12-knockdown-induced upregulation of SNAI1 ( Fig. 6b ). Consistent with these in vitro data, western blotting of lesional tissue lysates showed that phosphorylation of PKC, MEK and p38, and SNAI1 expression were increased on day 7 after injury, concomitant with reduced AKAP12 levels relative to those of normal tissues. These changes returned to basal levels by day 21 after injury, which was concomitant with the recovery in AKAP12 levels ( Fig. 6c ). These data show that AKAP12 regulates the expression of SNAI1 through the PKC/C-raf/MEK1 and p38 pathways. Figure 6: AKAP12 regulates SNAI1 expression through the non-Smad pathways of TGF-β1. ( a ) AKAP12-knockdown cells were serum starved for 6 h and then treated with TGF-β1 (10 ng ml −1 ) and/or RA (10 μM) for 20 min and 24 h. Inhibition of AKAP12 activated the PKC/C-raf/MEK1 and p38 pathways among the examined non-Smad pathways of TGF-β1. Activation of these pathways was closely correlated with SNAI1 expression. This data represent the results from independent three experiments. R, RA; T, TGF-β1; TR, co-treatment of TGF-β1 and RA; C, Cont; A, AKAP12. ( b ) Specific inhibitors for PKC, C-raf, MEK1 and p38 blocked the upregulation of SNAI1 induced by AKAP12 knockdown. After serum starvation for 24 h, inhibitors were added to AKAP12-knockdown ARPE-19 cells treated with TGF-β1 (10 ng ml −1 ) and RA (10 μM) for 24 h (mean±s.d., n =3, analysis of variance (ANOVA) followed by Tukey–Kramer test: * P <0.0005). GF 109203X (general PKC inhibitor): 5 μM, Bay 43-9006 (Raf-1 inhibitor): 1 μM, U0126 (MEK1 inhibitor): 10 μM, SB203580 (P38 inhibitor): 10 μM. ( c ) Lesional tissues from four mice per time point were collected and protein levels in the lesional tissue extracts were determined by western blot analysis. AKAP12 expression dynamically changed during the repair process. Phosphorylation of PKC, MEK1, p38 and SNAI1 expression had the opposite pattern to that of AKAP12 levels, similar to the in vitro data. Bands were quantified with Image J. AKAP12, SNAI1 and pan-PKC-P densities were normalized to that of α-tubulin. The densities of MEK-P and p38-P were normalized to that of total MEK and total p38, respectively (mean±s.d., n =4 mice per time point, ANOVA followed by Tukey–Kramer test: normal_* P <0.0005, ** P =0.003/PT 21_* P <0.0005, ** P =0.001). Full size image As the most important organ that regulates various activities of life, homeostasis of the CNS is directly connected to mental and physical abilities. Despite such importance, CNS tissue is vulnerable to external factors and exhibits poor regeneration after injury [44] . Therefore, it is thought that the CNS exhibits rapid defence and repair mechanisms to reduce damage from emergency conditions, which is unique when compared with those of other organs. In this respect, our results suggest that a balance of meningeal TGF-β1, RA and oxygen tension may constitute a stand-by mechanism that enables induction of EMT for rapid meningeal reconstruction after CNS injury. In this hypothesis, AKAP12 switches on and off this stand-by mechanism by responding to changing oxygen concentrations during the repair process. Under normal conditions, TGF-β1, RA and oxygen maintain meningeal AKAP12 expression and high levels of AKAP12 block TGF-β1-induced EMT. The Smad pathway is directly blocked by RA, and non-Smad pathways are indirectly inhibited by high levels of AKAP12 induced by both the RA/RARβ and the TGF-β1/Smad3 pathway ( Fig. 7a,d ). Immediately after CNS injury, hypoxia, caused by vessel damage, reduces AKAP12 levels by inhibiting RARβ expression, resulting in immediate EMT by de-repression of TGF-β1/non-smad/SNAI1 signalling pathways ( Fig. 7b,d ). In the later stages of repair, oxygen resupplied through neo-vessels restores AKAP12 levels and consequently, induces re-epithelialization of meningeal cells that have migrated to the lesional site by repressing TGF-β1/non-smad/SNAI1 signalling pathways. Finally, the meninges are reconstructed around the lesion ( Fig. 7c,d ). 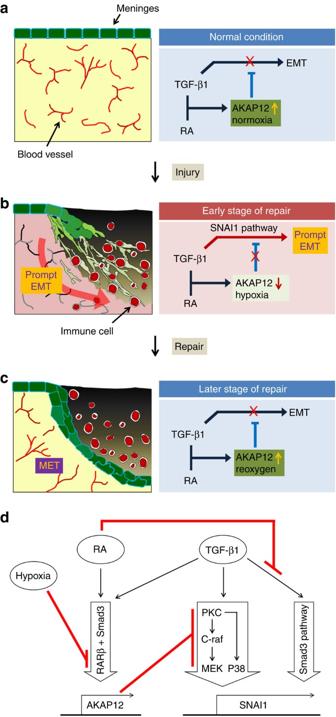Figure 7: Schematic model for prompt meningeal reconstruction and its molecular mechanism. (a) Under normal conditions, meningeal cells maintain a high level of AKAP12 because of the high concentrations of TGF-β1, RA and oxygen. AKAP12 maintains the epithelial properties of the meninges by inhibiting the TGF-β1 pathway. (b) Immediately after injury, hypoxia due to vessel damage de-represses the TGF-β1-SNAI1 pathway by suppressing the expression of AKAP12 resulting in meningeal cells’ EMT. Meningeal cells transited to the mesenchymal state by AKAP12 suppression invade into the site of the lesion. (c) At a later stage of repair, neo-microvessels formed by angiogenesis resupply oxygen to the site of the lesion. AKAP12 recovered by reoxygenation represses the TGF-β1-SNAI1 pathway, resulting in re-epithelialization of meningeal cells. (d) The diagram for the molecular mechanism of prompt meningeal reconstruction. Under co-treatment with RA and TGF-β1, the Smad pathway is directly blocked by RA, and non-Smad pathways are indirectly inhibited by high levels of AKAP12, the expression of which is induced by both RA and TGF-β1 under normoxic condition. In the hypoxic condition, AKAP12 expression is suppressed through RARβ repression. Then, the suppression of AKAP12 levels increases the level of SNAI1 by de-repression of the PKC/c-Raf/MEK1 and PKC/P38 pathways of TGF-β1, resulting in EMT. Figure 7: Schematic model for prompt meningeal reconstruction and its molecular mechanism. ( a ) Under normal conditions, meningeal cells maintain a high level of AKAP12 because of the high concentrations of TGF-β1, RA and oxygen. AKAP12 maintains the epithelial properties of the meninges by inhibiting the TGF-β1 pathway. ( b ) Immediately after injury, hypoxia due to vessel damage de-represses the TGF-β1-SNAI1 pathway by suppressing the expression of AKAP12 resulting in meningeal cells’ EMT. Meningeal cells transited to the mesenchymal state by AKAP12 suppression invade into the site of the lesion. ( c ) At a later stage of repair, neo-microvessels formed by angiogenesis resupply oxygen to the site of the lesion. AKAP12 recovered by reoxygenation represses the TGF-β1-SNAI1 pathway, resulting in re-epithelialization of meningeal cells. ( d ) The diagram for the molecular mechanism of prompt meningeal reconstruction. Under co-treatment with RA and TGF-β1, the Smad pathway is directly blocked by RA, and non-Smad pathways are indirectly inhibited by high levels of AKAP12, the expression of which is induced by both RA and TGF-β1 under normoxic condition. In the hypoxic condition, AKAP12 expression is suppressed through RARβ repression. Then, the suppression of AKAP12 levels increases the level of SNAI1 by de-repression of the PKC/c-Raf/MEK1 and PKC/P38 pathways of TGF-β1, resulting in EMT. Full size image These results provide a valuable insight into why the meninges maintains TGF-β1 expression even under normal conditions, in contrast to other epitheliums in which TGF-β1 expression is induced after injury [45] , [46] , and how the meninges retains epithelial properties despite the presence of TGF-β1, a major EMT-inducing factor. If pro-EMT factors are synthesized through a de novo pathway activated after CNS injury, achieving an immediate response will be difficult. Therefore, it is thought that the meninges maintains a stand-by state against emergencies through constant TGF-β1 expression. Simultaneously, meningeal RA may prevent the effects of TGF-β1 by inducing high levels of AKAP12 in conjunction with TGF-β1 and oxygen, consequently maintaining the epithelial properties of the meninges. The CNS has a high dependence on oxygen; therefore, oxygen concentrations are tightly regulated for proper function and homeostasis of the CNS [18] . Thus, vessel remodelling immediately occurs to replace impaired vessels after injury, and consequently, oxygen concentrations dynamically change during the repair process [47] . Such alterations in oxygen tension are important for tissue remodelling [48] . Furthermore, oxygen tension is rapidly changed by vascular state and has a direct effect on target molecules without requiring a specific receptor-mediated signalling cascade. Therefore, oxygen tension may control the immediate response after injury. Furthermore, oxygen tension is closely associated with the RA and TGF-β1 signalling pathways under physical and pathological conditions [49] , [50] . In this respect, we attempted to understand the process of prompt meningeal reconstruction in terms of the relationship between oxygen tension and the balance of RA and TGF-β1 signalling. We found that oxygen tension, which depends on vessel state, was closely associated with the transition between the epithelial and mesenchymal states of meningeal cells in vivo and that, although RA had an inhibitory effect on TGF-β1-induced EMT under normoxia, the inhibitory effect of RA was abolished under hypoxia in vitro ( Fig. 3 ). These results suggest that oxygen tension could be a regenerative microenvironment, which modulates reversibility of the meningeal state by regulating the balance between RA and TGF-β1 during prompt meningeal reconstruction. Finally, we identified AKAP12 as a candidate effector that could potentially modulate meningeal reconstruction, the expression of which was regulated by integrated upstream signals comprised of TGF-β1, RA and oxygen tension. In this study, we provide histological and in vitro evidence that suggests that AKAP12 regulates EMT/MET in meningeal cells during meningeal reconstruction. In a previous study, we compared the phenotypes of AKAP12 KO mice with wild-type mice after brain injury [26] . Although this previous study only focused on the functional aspects of the structure formed by AKAP12-positive cells surrounding the lesional site as a physical barrier, the in vivo data of the previous study strongly support the present in vitro data. In the previous study, the number of AKAP12-positive cells increased in the fibrotic scar surrounding the lesion at a late stage of repair. Since AKAP12-positive cells tightly trap immune cells with high levels of tight junction protein expression, the structure formed by the AKAP12-positive cells functions as a barrier to restrict inflammation in the fibrotic scar. Compared with wild-type mice, AKAP12 KO mice showed malfunction of the barrier structure with loss of the tight junction complex after injury, resulting in extended inflammation and more severe tissue damage. On the basis of serial observations in our injury model, it is thought that the barrier structure is a middle stage of the reconstruction process of the injured meninges. Reduced levels of tight junction proteins, epithelial markers of the barrier structure, in AKAP12 KO mice demonstrate that re-epithelialization of meningeal cells is abnormal during the later stages of repair, suggesting that AKAP12 is crucial for maintenance of epithelial properties in vivo , consistent with our in vitro study. Therefore, we propose that AKAP12 is a key factor that regulates EMT/MET in meningeal cells during meningeal reconstruction. Both Smad and non-Smad pathway were activated by TGF-β1, and SNAI1 induction by TGF-β1 has been traditionally linked to the canonical Smad pathway. However, non-Smad pathways that regulate TGF-β1-induced SNAI1 expression have recently been identified [51] , [52] , [53] , [54] . These studies reported an association between activation of PKC, MEK and p38 pathways and TGF-β1-induced SNAI1 expression similar to our results. Furthermore, Cao et al. [55] and Hoover et al. [56] reported that RA reduces TGF-β1-induced phosphorylation of Smad2/3, and Pendaries et al. [57] suggested that RAR blocks the formation of the Smad3/Smad4 complex by directly interacting with Smad3, suggesting that RA inhibits TGF-β1-induced Smad pathway activation. These previous studies strongly support the observation that AKAP12 regulates SNAI1 expression through the PKC/C-raf/MEK1 and PKC/p38 pathways (the non-smad pathways of TGF-β1) when TGF-β1-induced Smad pathway activation is inhibited by RA. Future studies will investigate how AKAP12 regulates the above pathways. Several previous studies provide valuable information for the investigation. It has been reported that the basic residue-rich binding domain of AKAP12 directly inhibits PKC activity [58] and that AKAP12, a scaffolding protein, blocks PKC activity by spatially separating PKC from its downstream factors [25] , [59] . Therefore, AKAP12 may regulate TGF-β1-induced PKC/C-raf/MEK1 and PKC/p38 pathway activity by binding to PKC, an upstream effector of these cascades, thereby inhibiting its activity. AKAP12 expression is primarily detected at the plasma membrane and along the cortical cytoskeleton in most cell types [60] . This expression pattern was also observed in the ex vivo -cultured meningeal tissue ( Fig. 1c ). Furthermore, PKC, a potential target of AKAP12, is activated at the plasma membrane. When activated by TGF-β1, the TGF-β1 type II receptor forms a complex with the TGF-β type I receptor to activate the transmembrane serine/threonine kinase activity of the TGF-β type I receptor. Then, activated TGF-β type I receptor triggers both signalling pathways by phosphorylating upstream components of Smad and non-Smad pathways [61] . On the basis of these parallel plasma membrane localizations, AKAP12 may be associated with TGF-β receptor complex signalling to upstream components of the PKC/C-raf/MEK and PKC-p38 pathways. Breakage of the meningeal barrier is a direct cause of CSF leakage, and patients with CSF leakage have a higher likelihood of intracerebral aerocele, meningitis and extended secondary damage related to malfunction of the meningeal barrier [5] , [6] . The duration of CSF leakage is an important factor when evaluating specific treatments (medication or surgical intervention) for meningeal barrier malfunction. Therefore, the degree of recovery after meningeal damage can be implied by levels of CSF leakage. CSF leakage occurs in 3% of closed head injuries, 9% of penetrating head injuries and 10–30% of basilar skull fractures [62] . Approximately, 80% of traumatic CSF leakage presents within 24–48 h after accident and 66% of post-traumatic CSF leakage ceases within 1 month [63] . Judging by these previous studies, much variation exists in the restoration time of the meningeal barrier. This variation is thought to stem from the diverse types and various degrees of damage that may occur during, for example, falls, motoring accidents or penetration. In the fixed PT condition described in Methods, 2 weeks are required before the reconstructed meninges restores its function as a physical barrier, without a large individual variation unlike human cases. Although we cannot completely exclude possible interspecies differences, control of the injury condition is expected to be the major reason for the disparity between animal models and human data. The recuperation period increases in accord with the scale of injury (illuminated diameter). Furthermore, when the diameter of the injury site was 2 mm or more, our model showed high individual variation in the recovery period and some mice exhibited cavities around the injury and failure of meningeal reconstruction. Furthermore, in mice younger than 5 weeks of age, we observed that PT induction largely increased the number of mice with injury site cavities and meningeal reconstruction failure. Similar to this observation, a recent clinical study showed that CSF leakage, haematoma and prolonged loss of consciousness increased the likelihood of paediatric readmission after medical treatment relative to that of adults [64] . These human data and observations in our injury model suggest that recovery of the impaired meningeal barrier is dictated by the severity of the CNS damage, and defective reconstruction of meningeal barrier may be more harmful in children than in adults. Therefore, further research is required to develop manualized treatments targeting meningeal barrier function according to the severity of the CNS injury and the age of patient. Interestingly, TGF-β1, RA and oxygen tension, which regulate the AKAP12 level in our stand-by EMT model, are regulatory factors of EMT during development, cancer metastasis and organ fibrosis. TGF-β1 is an important EMT-inducing factor [11] , [65] , and RA may inhibit EMT during heart development [66] and lung fibrosis [67] . Furthermore, a hypoxic microenvironment upregulates pathological EMT by inducing SNAI1 expression [68] . As our results are in agreement with these previous studies, there may be connecting links among these previous studies. Therefore, extended studies are warranted to examine whether the AKAP12-mediated EMT/MET regulatory mechanisms herein also apply to development, cancer metastasis and organ fibrosis. Animals and photothrombosis Animal experiments were approved by the Committee for Care and Use of Laboratory Animals at Seoul National University, according to the Guide for Animal Experiments edited by the Korean Academy for Medical Sciences. Male C57BL/6 mice (age: 6–8 weeks, weight: 23–25 g) were used for photothrombosis [69] . Under anaesthesia, rose bengal (Sigma, 10% solution, 0.1 ml per 25 g of body weight) was circulated for 5 min via tail vein injection. After scalp incision, the skull was illuminated with a cold light source (Zeiss FL1500 LCD, 150 W, 1 mm diameter) for 20 min. The position of the optic centre was 2.5 mm to the left and 2.5 mm to the back of the bregma. The scalp was sutured, and mice were allowed to wake from anaesthesia. Cell culture and related procedures The human retinal pigment epithelial cell line, ARPE-19, was cultured in DMEM/F12 with 10% fetal bovine serum (FBS). The adenocarcinomic human alveolar basal epithelial cell line, A549, was cultured in DMEM with 10% FBS. For meningeal ex vivo culture, meningeal tissues were isolated from the brains of postnatal day 3 mice. After mild digestion with trypsin EDTA solution (Gibco, 0.25%), meningeal tissues were attached to poly- L -lysine-coated labware and cultured in DMEM with 10% FBS. ARPE-19 and A549 cells were purchased from American Type Culture Collection. Immunofluorescence Under anaesthesia, mice were perfused with 0.1 M phosphate-buffered saline (pH 7.4) and fixed with 4% paraformaldehyde. Isolated brains were dehydrated with serial gradients of sucrose at 4 °C. Cryostat sections of 10-μm thicknesses were attached to gelatin-coated slides and 30-μm-thick sections were stored in preservation solution for free-floating staining. For staining of epithelial markers in the meninges, brains were frozen immediately after extraction and 10-μm-thick cryostat sections were fixed with 4% paraformaldehyde for 15 min at room temperature (RT). For staining of RARβ and SNAI1, brains were frozen immediately after extraction and 8-μm-thick cryostat sections were fixed with 100% methanol for 1 h at −20 °C. Cells were fixed with 100% ethanol (4 °C, 30 min), following gentle washing with 100% acetone (resting temperature, 1 min), and blocked with 3% skim milk in phosphate-buffered saline at RT for 30 min. Samples were stained with primary antibodies against AKAP12 (I.H. Gelman, Roswell Park Cancer Institute, 1:500), ERTR7 (Abcam, 1:200), E-cadherin (BD Biosciences, 1:300), CD31 (BD Biosciences, 1:100), occludin (Invitrogen, 1:200), ZO-1 (Invitrogen, 1:200), GFAP (Dako, 1:1,000), fibronectin (Dako, 1:1,000), α-SMA (Dako, 1:100), RALDH2 (Santa Cruz, 1:100), TGF-β1 (Santa Cruz, 1:100), RARβ (Novus, 1:200) and SNAI1 (Novus, 1:200) overnight at 4 °C, followed by Alexa 488, 546 and 350 (Invitrogen, 1:3,000) secondary antibodies at RT for 1 h. A Zenon IgG Labeling Kit (Invitrogen) was used for double staining. Nuclear staining was performed with Hoechst 33342 (Molecular Probes). An ApoTome microscope (Carl Zeiss, Axiovert M200) and a confocal microscope (Carl Zeiss, LSM700) were used for image analysis. Western blotting Lesional tissues were homogenized and cell samples were lysed in a buffer (20 mM Tris-HCl (pH 7.5), 150 mM NaCl, 1 mM Na 2 EDTA, 1 mM EGTA, 1% Triton, 2.5 mM sodium pyrophosphate, 1 mM beta-glycerophosphate, 1 mM Na 3 VO 4 , 1 μg ml −1 leupeptin and protease inhibitor cocktail). For detection of HIF-1α and SNAI1, cells were frozen with liquid nitrogen and then lysed in whole cell extraction buffer (10 mM HEPES (pH 7.9), 400 mM NaCl, 0.1 mM EDTA, 5% glycerol, 2.5 mM sodium pyrophosphate, 1 mM beta-glycerophosphate, 1 mM Na 3 VO 4 , 1 μg ml −1 leupeptin and protease inhibitor cocktail). Immunoblotting was performed with primary antibodies against AKAP12 (Santa Cruz, 1:6,000), RARβ (Santa Cruz, 1:1,000), α-tubulin (InnoGenex, 1:8,000), E-cadherin (BD, 1:3,000), HIF-1α (BD, 1:3,000), ZO-1 (Invitrogen, 1:3,000), occludin (Invitrogen, 1:3,000), α-SMA (Dako, 1:1,000), SNAI1 (Cell Signaling, 1:500), pan-phospho-PKC (Cell Signaling, 1:1,000), phospho-C-raf (Cell Signaling, 1:1,000), C-raf (Cell Signaling, 1:3,000), phospho-MEK1 (Cell Signaling, 1:1,000), MEK1 (Cell Signaling, 1:3,000), phospho-p38 (Cell Signaling, 1:1,000), p38 (Cell Signaling, 1:3,000), phospho-Smad2 (Cell Signaling, 1:1,000), phospho-Smad3 (Cell Signaling, 1:1,000) and Smad2/3 (Cell Signaling, 1:6,000). The images of the full blots are presented in Supplementary Fig. 6 . Transfection and reverse transcription PCR A human RARβ plasmid, pCMV tag2b_flag, was transfected into ARPE-19 cells with polyethylenimine (Sigma). Each siRNA was transfected into ARPE-19 cells using Oligofectamine (Invitrogen) and A549 cells with DharmaFECT duo (Dharmacon) according to the manufacturers’ instructions. RNA was extracted with Trizol reagent (Invitrogen) and complementary DNA was obtained by reverse transcription. Sequences for siRNA and primers are presented in Supplementary Table 1 . Images of the full DNA gel are presented in Supplementary Fig. 6 . Data analysis and statistics Bands were quantified with Image J and normalized to the density of glyceraldehyde-3-phosphate dehydrogenase and α-tubulin. Statistical analysis was performed using analysis of variance followed by post hoc analysis with the Tukey–Kramer test for multiple comparisons. P <0.05 was considered statistically significant. How to cite this article: Cha, J.-H. et al. Prompt meningeal reconstruction mediated by oxygen-sensitive AKAP12 scaffolding protein after central nervous system injury. Nat. Commun. 5:4952 doi: 10.1038/ncomms5952 (2014).